Mutual adaptation of a membrane protein and its lipid bilayer during conformational changes The structural elucidation of membrane proteins continues to gather pace, but we know little about their molecular interactions with the lipid environment or how they interact with the surrounding bilayer. Here, with the aid of low-resolution X-ray crystallography, we present direct structural information on membrane interfaces as delineated by lipid phosphate groups surrounding the sarco(endo)plasmic reticulum Ca 2+ –ATPase (SERCA) in its phosphorylated and dephosphorylated Ca 2+ -free forms. The protein–lipid interactions are further analysed using molecular dynamics simulations. We find that SERCA adapts to membranes of different hydrophobic thicknesses by inducing local deformations in the lipid bilayers and by undergoing small rearrangements of the amino-acid side chains and helix tilts. These mutually adaptive interactions allow smooth transitions through large conformational changes associated with the transport cycle of SERCA, a strategy that may be of general nature for many membrane proteins. Membrane proteins are integral parts of biomembranes, working as gatekeepers of biological transport and signalling processes. Their function is crucially dependent on the general physical properties of the surrounding lipid bilayer, such as hydrophobic thickness, phase and viscosity [1] , [2] , [3] , [4] , [5] , as well as on specific interactions between the protein and the membrane components [5] , [6] . Protein crystallography has in recent years succeeded in providing detailed structures of a number of membrane proteins, and in some cases also of specific lipid contacts [7] , [8] , [9] , [10] , [11] , [12] . However, little structural information is available on how membrane proteins are actually positioned within the lipid bilayer, and how the interactions with the membrane change in response to, or as a means of, functional transitions. The issue is complicated by the fact that it is rarely possible to achieve imaging of membrane proteins and a lipid bilayer environment at the same time, except for a few targets showing unusually favourable properties such as bacteriorhodopsins and aquaporins [8] , [10] , [12] . If the protein structure is known, it has for several years been possible to model the protein in a bilayer environment with molecular dynamics (MD) simulations. This has, however, been carried out without the possibility to validate the modelling by direct imaging. Here we present an analysis of the interactions between a membrane protein and the phospholipid bilayer in which it is embedded, based on a combination of X-ray data and MD simulations. The membrane protein is the sarco(endo)plasmic reticulum Ca 2+ –ATPase (SERCA), a P-type ATPase that transports Ca 2+ ions from the cytoplasm into the sarcoplasmic reticulum (SR) store to terminate muscle contraction. On the basis of a vast amount of experimental data on SERCA, much is known about the structure and function of this transport protein. Nevertheless, some structural aspects remain relatively unexplored, such as the interplay of SERCA with its immediate lipid environment as well as the effect of the general physical properties of the lipid bilayer [5] , [13] , [14] . For an analysis of these effects, we took advantage of SERCA crystals grown from purified SR membranes, which are solubilized by octaethyleneglycol dodecyl monoether (C 12 E 8 ) detergent in a manner that retains the functional properties of the ATPase [15] , [16] , [17] . Diffracting crystals composed of stacked two-dimensional (2D) layers [18] with large lipid–detergent content are obtained, and for two functional states, we obtain direct structural information on the phospholipids present as bilayers in the crystals. Encouragingly, these observations are consistent with independent MD simulations of SERCA in similar lipid–detergent bilayers. We then proceed to analyse the interactions of SERCA with lipid bilayers of different thicknesses. From the simulations, we explain why an apparent mismatch between the hydrophobic thickness of the bilayer and the membrane-embedded sector of SERCA [5] is required to allow sufficient freedom for the protein to undergo large conformational changes associated with Ca 2+ transport across the SR membrane. Protein position in the bilayer Owing to the crystal packing of SERCA molecules as stacked 2D crystals with significant lipid content [18] and to unaccounted features in electron density maps, we wondered whether crystallographically ordered bilayers could be visualized by means of the scattering from primarily the electron-dense lipid phosphate groups. Low-resolution X-ray diffraction data for crystals of the Ca 2+ -free and dephosphorylated enzyme, the so-called E2 form, stabilized by the inhibitor debutanoyl thapsigargin (dBTG) were therefore carefully collected. 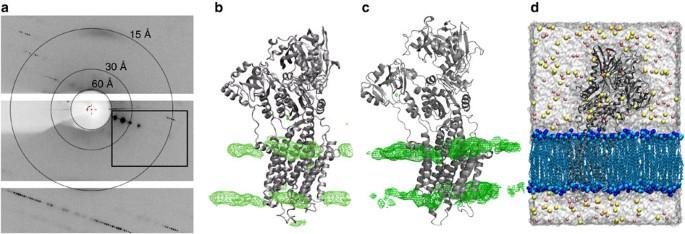Figure 1: Initial experimental observation and MD setup. (a) X-ray diffraction image (cropped) from the SERCA E2 crystal. Resolution rings are indicated, and broad low-resolution Bragg reflections with high intensity are indicated by a box. (b) The SERCA E2 crystal structure (PDB accession code 2YFY) with experimental difference electron density map (Fobs−Fcalc) calculated at 60–8 Å resolution and contoured at 2.6 σ is shown in green mesh. (c) Model-based difference electron density map (Fcalc (protein+lipid/detergent)−Fcalc (protein)) calculated at 60–8 Å resolution and contoured at 2.2 σ. The model is based on an MD simulation of SERCA in a POPC/detergent bilayer. (d) System setup for MD simulations of SERCA in bilayer environments; in this example, a POPC bilayer is shown in blue and SERCA by a schematic cartoon representation in dark grey. Potassium and chloride ions are shown as spheres in light pink and yellow, respectively, and water molecules by light grey surface (hydrogen atoms are omitted from the figure). Several of these reflections displayed very broad peak profiles with high intensity, as depicted in Figure 1a , indicating semiordered features in the crystal. By inclusion of nearly complete low-resolution data in the Fourier synthesis, valuable structural information concerning the position of SERCA as an integral membrane protein in a membrane was indeed obtained. As seen from Figures 1b and 2a , our data revealed electron density features outside the protein, in positions corresponding to the hydrophobic/hydrophilic interface expected of membrane bilayers. For a different functional state of the enzyme, the Ca 2+ -free, phosphorylated form called E2P, deposited data (PDB 3B9B [19] ) used for calculations of low-resolution electron density maps revealed similar features ( Fig. 2a ). Figure 1: Initial experimental observation and MD setup. ( a ) X-ray diffraction image (cropped) from the SERCA E2 crystal. Resolution rings are indicated, and broad low-resolution Bragg reflections with high intensity are indicated by a box. ( b ) The SERCA E2 crystal structure (PDB accession code 2YFY) with experimental difference electron density map ( F obs − F calc ) calculated at 60–8 Å resolution and contoured at 2.6 σ is shown in green mesh. ( c ) Model-based difference electron density map ( F calc (protein+lipid/detergent) − F calc (protein) ) calculated at 60–8 Å resolution and contoured at 2.2 σ. The model is based on an MD simulation of SERCA in a POPC/detergent bilayer. ( d ) System setup for MD simulations of SERCA in bilayer environments; in this example, a POPC bilayer is shown in blue and SERCA by a schematic cartoon representation in dark grey. Potassium and chloride ions are shown as spheres in light pink and yellow, respectively, and water molecules by light grey surface (hydrogen atoms are omitted from the figure). 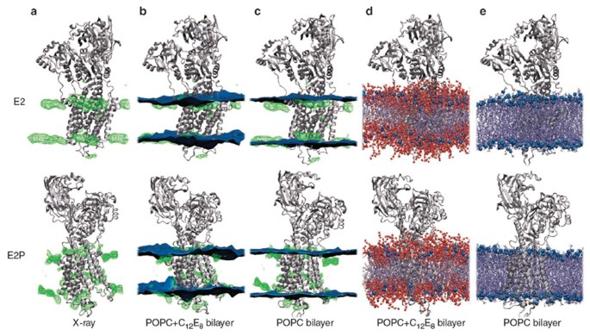Figure 2: Membrane low-resolution electron density compared with MD simulations of SERCA in the E2 and E2P conformations. Protein structure is shown in grey ribbon. (a) Crystal structures of SERCA with low-resolution electron densities from the same crystal in green mesh (60–8 Å resolution, 2.6 σ contour for E2; 30–8 Å resolution, 2.0 σ contour for E2P). (b) Average protein structure together with a blue surface representing the average positions of phosphorus atoms in the bilayer leaflets, calculated from a 50-ns MD simulation of SERCA in a bilayer mimicking crystal conditions. Low-resolution electron densities are shown in green mesh as ina. (c) Average protein structure together with a blue surface representing the average positions of phosphorus atoms in the bilayer leaflets, calculated from a 50 ns MD simulation of SERCA in a pure POPC bilayer. Low-resolution electron densities in green mesh as inaandb. Discrepancies are evident. (d) Snapshot after 50 ns of the MD simulation described inb. Detergent is shown in pink with red oxygen atoms and lipids in light blue with blue phosphorus atoms. (e) Snapshot after 50 ns of the MD simulation described inc, lipids shown as ind. Full size image Figure 2: Membrane low-resolution electron density compared with MD simulations of SERCA in the E2 and E2P conformations. Protein structure is shown in grey ribbon. ( a ) Crystal structures of SERCA with low-resolution electron densities from the same crystal in green mesh (60–8 Å resolution, 2.6 σ contour for E2; 30–8 Å resolution, 2.0 σ contour for E2P). ( b ) Average protein structure together with a blue surface representing the average positions of phosphorus atoms in the bilayer leaflets, calculated from a 50-ns MD simulation of SERCA in a bilayer mimicking crystal conditions. Low-resolution electron densities are shown in green mesh as in a . ( c ) Average protein structure together with a blue surface representing the average positions of phosphorus atoms in the bilayer leaflets, calculated from a 50 ns MD simulation of SERCA in a pure POPC bilayer. Low-resolution electron densities in green mesh as in a and b . Discrepancies are evident. ( d ) Snapshot after 50 ns of the MD simulation described in b . Detergent is shown in pink with red oxygen atoms and lipids in light blue with blue phosphorus atoms. ( e ) Snapshot after 50 ns of the MD simulation described in c , lipids shown as in d . Full size image However, as the bilayers in the crystals contain an appreciable amount of detergent [18] , the question can be raised as to whether the detergent will affect the membrane lipids and the structure of the protein [20] , [21] . We therefore proceeded to analyse the expected behaviour of SERCA by MD simulations, both in a pure palmitoyl-oleoyl phosphatidylcholine (POPC) lipid bilayer (mimicking a native membrane) and in a bilayer with both C 12 E 8 detergents and POPC lipids randomly distributed in a 2:1 molar ratio (to mimic the crystal conditions with an approximate 1:30:80 protein:lipid:detergent molar ratio [18] ). The average protein structures and the average topography of bilayer interfaces, determined from the position of the phosphorus atoms in the bilayer leaflets, were computed on the basis of these simulations ( Fig. 2b,c ). If the models are reliable and consistent, the average bilayer interfaces, obtained from the unbiased simulations with inclusion of detergent, should overlay with the low-resolution electron densities observed from the crystal structures. This was indeed the case: the MD simulations of the crystal-mimicking system clearly match the experimental structures both with respect to the membrane thickness and the orientation of the protein relative to the bilayer ( Fig. 2b ). This represents a clear illustration of how membrane proteins in this type of crystals are in fact surrounded by a bilayer environment. Furthermore, it provides a strong validation of the MD procedure and invites further modelling and analysis of the interactions of SERCA with different types of lipid bilayers. Detergent effect on membrane and protein structure From the MD simulations in a pure POPC membrane versus a detergent-containing membrane ( Fig. 2c,e versus b,d ), we can now directly analyse the effect of the C 12 E 8 detergent on the structure of the bilayer surrounding the membrane protein. Because of its amphipathic structure with a long polyether 'head-group' and short hydrophobic tail, the position and orientation of the detergent molecules along the membrane normal is not as restricted as it is for the lipid molecules. This allows for a very flexible amphipathic environment around the protein in the mixed detergent bilayer, at which the lipid molecules also can occupy a broader distribution along the membrane normal without significant energetic cost. Thereby, the local requirements for favourable interactions at the protein surface are well accommodated inside the detergent-containing membrane. The more diffuse membrane interface resulting from the detergent-containing bilayer is also clearly visualized by the distribution of the carbonyl oxygen atoms of the glycerol linkage in the POPC lipids along the membrane normal ( Supplementary Fig. S1 ). In addition, the density of detergent head-group oxygen atoms, although highest at the membrane interfaces, is seen to be non-zero all through the membrane. This illustrates that the detergent molecules are not strictly associated with one of the two leaflets, but are capable of permeating through the membrane in accordance with experimental evidence [22] . To evaluate whether the protein structure adapts differently to the detergent-containing bilayer compared with a pure lipid bilayer, the average structures obtained in the two environments were compared. For both the E2 and the E2P conformations, the transmembrane parts of the structures observed in the two environments were very similar, having Cα-root mean square deviation (RMSD) values below 1.5 Å ( Supplementary Tables S1 and S2 ). To assess whether the protein structures had changed compared with the original crystal structures, the average structures were also compared to these, and again the Cα-RMSD values were below 1.5 Å ( Supplementary Tables S1 and S2 ). Thus, it appears that the protein structure is only slightly affected by the detergent environment, consistent with a functional integrity. [15] Hydrophobic thickness of SERCA Assuming that the location of tryptophan and basic residues indicate putative membrane interfaces, it has been noted that SERCA displays a surprisingly narrow hydrophobic thickness of 21–24 Å [5] , [23] ( Supplementary Fig. S2 and Supplementary Note 1 ). SERCA, however, displays maximum activity when embedded in membranes with hydrophobic thicknesses around 30 Å [13] , [24] , just as seen for many other membrane proteins [14] , [25] , [26] , [27] , [28] , [29] . To inspect the structural basis and possible functional implications of this apparent mismatch, which has also been noted to exist for other membrane proteins [5] , [30] , we performed MD simulations of SERCA in the E2 and E2P conformations inserted in three pure lipid bilayers ( Supplementary Fig. S3 ), namely dimyristoleoyl phosphatidylcholine (C14:1 9c, C14:1 9c), referred to as (di-C14:1)PC, POPC (C16:0, C18:1 9c), and stearoyl gadoleyl phosphatidylcholine (C18:0, C20:1 9c), referred to as SGPC. From our simulations, the estimated hydrophobic thicknesses of these bilayers are 23, 29 and 32 Å, respectively. For each simulation, the average structure of the protein and the average bilayer leaflet surfaces were calculated ( Fig. 3 and Supplementary Fig. S4 ). Remarkably, we find that most of the potentially unfavourable hydrophobic/hydrophilic interactions are avoided, irrespective of changes in the average hydrophobic thickness of the particular membrane. The membrane contributes to the adaptation by local deformations of the bilayer hydrophobic/hydrophilic interface, observed as deviations from average positions in the order of ±4 Å around the protein ( Supplementary Fig. S4 ). These changes are accompanied by structural adjustments of the protein consisting of side-chain rotations ( Supplementary Fig. S5 ) and small helix tilt changes ( Supplementary Fig. S6 ). 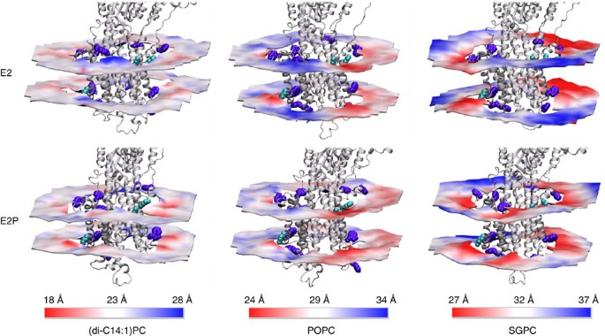Figure 3: Hydrophobic matching for SERCA in the E2 and E2P conformations. Average structures of SERCA are shown in grey ribbons. Tryptophan residues (except residues 272 and 794) are shown in blue spheres, and basic residues in the membrane region are shown in cyan spheres. Average hydrophobic/hydrophilic interfaces, shown as surfaces, are calculated from MD simulations of SERCA positioned in the different membrane environments. The membrane environments are as follows: (di-C14:1)PC lipids (C14:1, C14:1), POPC lipids (C16:0, C18:1) and SGPC lipids (C18:0, C20:1), with hydrophobic thicknesses of 23, 29 and 32 Å, respectively. The membrane interface is defined by the carbonyl oxygen atoms in the lipid glycerol linkage and coloured based on deviation from the average hydrophobic thickness along the membrane normal. As can be seen from Figure 3 , the membrane deformations do not lead to a uniform thinning of the thicker membranes (POPC and SGPC) as depicted in schematic biophysical models of membrane protein/lipid mismatch [5] , [31] . Rather, thinning is observed locally, in particular to accommodate hydrophilic side chains where present. To rationally explain why POPC is observed to provide a more optimal environment for SERCA than (di-C14:1)PC, we examined the surface-exposed residues in more detail ( Fig. 4 ). In the POPC bilayer, the overall hydrophobic–hydrophilic requirements of the SERCA protein surface are fulfilled the best. This is achieved, in part, by 'snorkelling' of the buried basic side chains towards the polar interface, combined with local deformations at the membrane interface to avoid the charged residues from being trapped in the hydrophobic part of the thicker membrane. For (di-C14:1)PC, the situation is very different: a total of around ten hydrophobic amino-acid residues (being buried in the hydrophobic part of the POPC bilayer, mainly at the luminal side) are exposed to the polar head-group region of the (di-C14:1)PC bilayer in both the E2 and E2P conformations. Hence, the short-chained (di-C14:1)PC lipids surround the membrane domain similar to a straitjacket that prevents the rotational and translational movements of the transmembrane helices associated with conformational changes, which would lead to further exposure of hydrophobic residues. Figure 3: Hydrophobic matching for SERCA in the E2 and E2P conformations. Average structures of SERCA are shown in grey ribbons. Tryptophan residues (except residues 272 and 794) are shown in blue spheres, and basic residues in the membrane region are shown in cyan spheres. Average hydrophobic/hydrophilic interfaces, shown as surfaces, are calculated from MD simulations of SERCA positioned in the different membrane environments. The membrane environments are as follows: (di-C14:1)PC lipids (C14:1, C14:1), POPC lipids (C16:0, C18:1) and SGPC lipids (C18:0, C20:1), with hydrophobic thicknesses of 23, 29 and 32 Å, respectively. The membrane interface is defined by the carbonyl oxygen atoms in the lipid glycerol linkage and coloured based on deviation from the average hydrophobic thickness along the membrane normal. 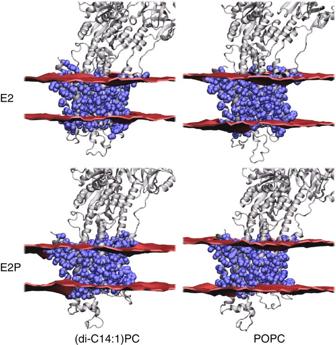Figure 4: Membrane coverage of hydrophobic residues. Average structures of SERCA from MD simulations of the E2 and E2P conformations in (di-C14:1)PC and POPC bilayers are shown in grey ribbon. Hydrophobic residues covered by the POPC membrane are shown in blue spheres. The average bilayer interfaces, as defined by the carbonyl oxygen atoms of the lipids, are shown in red. Full size image Figure 4: Membrane coverage of hydrophobic residues. Average structures of SERCA from MD simulations of the E2 and E2P conformations in (di-C14:1)PC and POPC bilayers are shown in grey ribbon. Hydrophobic residues covered by the POPC membrane are shown in blue spheres. The average bilayer interfaces, as defined by the carbonyl oxygen atoms of the lipids, are shown in red. Full size image Our refined analysis of the two Ca 2+ -free conformations of SERCA presented here demonstrates the importance and added value of including low-resolution data for calculation of electron density maps to explore the interactions of the protein with the surrounding lipid bilayer. We anticipate that many crystal structures of the so-called type I (stacked 2D crystals) may in fact, by closer analysis, show similar bilayer features as demonstrated here. At the same time, our approach invites further development of density modification procedures for membrane proteins so that these can be analysed by at least three levels of 'bulk solvent' handled simultaneously: the aqueous solvent (standard bulk solvent), the bilayer interfaces (as revealed in this study) and the hydrophobic core of the bilayers (with a supposedly lower average density compared with the other two). From our simulations, it appears that the apparent hydrophobic mismatch between the protein and the lipid bilayer results in the formation of localized adaptation characterized by local deformations of the bilayer and small rearrangements of amino-acid side chains and helix tilts. Energetically, these structures can be assumed to balance the opposing forces that arise from changes in the lipid and/or protein component to minimize the hydrophobic/hydrophilic mismatch. However, the opposing forces cannot completely correct the mismatch in the thin (22–23 Å) (di-C14:1)PC membranes, resulting in defective ATPase function. We note that, although the transmembrane domain of SERCA seems to be adequately shielded by a detergent-containing bilayer of ~25 Å thickness, in the absence of detergent, the enzyme requires a larger hydrophobic span of ~30 Å. This is needed to decrease the energy barriers to allow the smooth transition between the conformational changes associated with the various steps of the catalytic cycle. This requirement cannot be fulfilled for thin membranes, whereas for too thick membranes the hydrophobic coverage (mismatch) becomes too pronounced for proper interaction between the protein and the lipids. The straitjacket effect of a thin membrane is consonant with functional defects of SERCA in (di-C14:1)PC bilayers, namely, a severely reduced rate of dephosphorylation of the ATP-phosphorylated intermediate E2P, and binding and transport of only one rather than two Ca 2+ ions per ATPase cycle [13] , [24] . The conformational changes between E1 (Ca 2+ -bound) and E2 (Ca 2+ -free) states implicate relative up–down translocations of transmembrane helices in the order of 5 Å [32] , [33] . In lipid bilayers of medium thickness, as e.g. POPC, the flexible and adaptive protein/lipid interface may therefore ensure that the conformational changes associated with the functional cycle can occur without significant energy barriers caused by hydrophobic/hydrophilic mismatches and as such liberate the transition kinetics. In support of this model, the estimates of free-energy changes for membrane insertion (Δ G transfer ) listed by the Orientations of Proteins in Membranes (OPM) database [30] indicate that all known SERCA structures, representing five different conformations of the functional cycle, display comparable values (−60 to −70 kcal mol −1 ). It is tempting to generalize our model of an adaptive and flexible protein–membrane interface to transporters as a whole, for which energy barriers of conformational changes between their different transport states are rate limiting. Different criteria may, however, apply for proteins that undergo conformational change under a strict control, such as signal-transducing receptors or transporters, for which a specific activation barrier might be important as a point of functional regulation. We foresee that the experimental and theoretical approaches as depicted here will go hand in hand to further explore the dynamics of biomembranes. Protein purification SERCA (isoform 1a) was isolated from SR vesicles of rabbit fast-twitch skeletal muscles and purified by treatment with a low concentration of deoxycholate before solubilization [34] . For crystallization, the ATPase was solubilized by a minimal amount of the detergent C 12 E 8 to an approximate 1:3 ratio of native membrane lipids and the detergent. The protein buffer consisted of 100 mM 3-( N -morpholino)propanesulfonic acid (pH 6.8) with 20% (v/v) glycerol, 80 mM KCl, 2 mM ethylene glycol tetra-acetic acid, 1 mM phosphomethylphosphonic acid adenylate ester (AMPPCP) and 3 mM MgCl 2 . The solubilization was performed in the presence of appropriate stabilizers and structural analogues, as described below. The resulting protein-bilayer topology is described in the Supplementary Methods . Crystallization and X-ray data collection Structure factors and coordinates for the E2–BeF 3 − structure, corresponding to the E2P phosphorylated state of SERCA with luminal orientation of the cation-binding sites (PDB 3B9B [19] ), were used for low-resolution electron density map calculations. To obtain an E2 structure for high- and low-resolution analysis, cocrystallization of SERCA with 1 mM AMPPCP and 125 μM dBTG was performed using vapour diffusion in hanging drops in 24-well crystallization trays. The protein sample was centrifuged in a Beckmann TLA-110 rotor (Beckmann) at 50.000 r.p.m. before use. Drops were composed of 2-μl reservoir solution plus 2-μl protein solution with a protein concentration of typically 10 mg ml −1 . Optimal conditions for crystallization were established at 4 °C with reservoirs containing 10% glycerol, 17% polyethylene glycol 6,000, 0.2 M NaCl and 6% 2-methyl-2,4-pentanediol. Crystals grew to a size of ~200×200×25 μm within a week. Crystals were equilibrated for 10–45 s in a protein-free solution composed of the reservoir solution with glycerol added to 25% (v/v) for the purpose of cryoprotection. They were then mounted in LithoLoops (Molecular Dimensions) that had been bent 90° to allow rotation along a nearly 600 Å long c -axis defining the thin dimension of the square plate crystals, and flash cooled in liquid nitrogen. A data set was collected at the Swiss Light Sources (SLS, Paul Scherrer Institute, Villigen) beamline X06SA on a Pilatus 6M detector (Pilatus) at a temperature of 100 K and a wavelength of 1.0718 Å. A total of 360 images were recorded with an oscillation range of 0.5°, showing no signs of radiation-mediated decay. Reflections at 60–3.1 Å resolution data were recorded in a single pass, taking advantage of the very large dynamic range (20 bits), low point spread and large area of the Pilatus 6M detector (Pilatus). Data processing and structure determination Data were scaled and merged using XDS [35] . No spurious diffraction features were observed that would disqualify the use of low-resolution data in the Fourier syntheses to derive electron density maps. The structure was determined by molecular replacement applying PDB 2C8K [33] as a search model and using Phaser [36] . Model building was performed in Coot [37] and crystallographic model refinement in Phenix [38] with TLS groups corresponding to each domain in SERCA. The coordinates of the energy-minimized inhibitor, dBTG, were obtained using the Dundee PRODRG server [39] , and restraints for the ligand were calculated using Refmac5 [40] . Statistics for data collection and processing are shown in Table 1 . The inclusion of low-resolution data improved the imaging of electron density features appearing as bilayers in the crystal. Further discussion on the use of low-resolution data can be found in the Supplementary Methods . Table 1 Data collection and refinement statistics. Full size table MD simulations setup X-ray structures of SERCA, corresponding to the E2 and the E2P forms, respectively, were used as starting structures for the protein. For the E2 conformation, a structure for a similar crystal form with a nortrilobolide inhibitor, refined at a higher resolution, was applied (PDB 3NAL [41] ). This structure has a Cα-RMSD of 0.5 Å to the E2 crystal structure reported here. The inhibitor and a magnesium ion were deleted, whereas the protein together with a bound potassium ion and water molecules were used for further system setup. The E2P form was based on the PDB entry 3B9B [19] . The magnesium ion located in the luminal exit pathway of the E2–BeF 3 − structure was deleted, and the sodium ion present in the cytosolic ion-binding site was changed to a potassium ion. The BeF 3 − complex was changed to a proper phosphorylation of the carboxylate side chain of Asp351 by changing the beryllium atom into phosphorus and the fluoride atoms into oxygen. The magnesium ion coordinated by BeF 3 − was left unchanged and was used for further system setup together with the crystallographic water molecules. Protonation states of ionizable side chains were based on pK a prediction by PROPKA [42] , [43] and by manual inspection, and were found to be robust in modelling studies (unpublished). In the empty Ca 2+ ion-binding sites, Glu309, Glu771 and Glu908 were protonated, and for the E2 structure, Glu703 was additionally protonated. A disulphide bond was formed between cysteine residues 876 and 888. A POPC membrane patch of 115×125 Å was generated using the Membrane Builder available in VMD [44] . A discussion on the POPC membrane model of the SR membrane can be found in the Supplementary Methods . The two protein structures were initially oriented in the membrane as proposed by the OPM database [30] . The systems were solvated using the Solvate package in VMD [44] to produce a simulation box with dimensions 115×125×163 Å 3 . Finally, the systems were ionized with K + and Cl − ions to neutralize the overall charge of the system and to yield an ionic concentration of 0.2 M using the ionization plug-in tool in VMD. The final system setup used for simulation of the E2 state in a POPC bilayer is shown in Figure 1d . Setups with different bilayer compositions ( Supplementary Fig. S3 ) were constructed from the setups with POPC bilayer, as described in the Supplementary Methods . This resulted in setups with four different bilayer environments for each SERCA conformation, namely, a pure (di-C14:1)PC bilayer ((C14:1 9c, C14:1 9c)), a pure SGPC bilayer ((C18:0, C20:1 9c)), a pure POPC bilayer ((C16:0, C18:1 9c)) and a bilayer with a mixture of POPC lipids and C 12 E 8 detergent molecules in the ratio of 1:2. See Supplementary Methods for a discussion of the validity of a random mixture of detergent and lipids in the bilayer. MD simulation protocol MD simulations were performed using the NAMD 2.6 program [45] , [46] , applying the TIP3P water model [47] . The CHARMM27 force field [48] was applied for the simulations; including the CMAP correction [49] for the protein backbone dihedral angles. In addition to these standard parameters, parameters for non-standard residues were added. Parameters for the dianionic phosphoaspartate were adapted from Damjanović et al . [50] Parameters for the detergent molecule, C 12 E 8 , were assembled from the CHARMM27 lipid parameters and the CHARMM ether parameters [51] , [52] as outlined in the Supplementary Methods and Supplementary Tables S3-S5 . Periodic boundary conditions were adopted. The long-range electrostatic interactions were handled with the PME method [53] with a maximum grid spacing of 1 Å. For short-range, non-bonded interactions, a cutoff of 12 Å was utilized, with the switching function starting at 10 Å. The pair list, with a cutoff of 14 Å, was updated every 20 time steps. The systems were minimized in 15,000 steps and the lipid tails (from carbonyl carbon atoms and down) were equilibrated for 0.5 ns, whereas the rest of the system was fixed. This so-called melting of the lipid tails was performed in the NVT ensemble with a temperature of 310 K. Langevin dynamics with a damping coefficient of 0.1 ps −1 was applied for controlling the temperature. Subsequently, 2 ns of equilibration was performed in the NPT ensemble with a temperature of 310 K controlled by Langevin dynamics with a damping coefficient of 0.5 ps −1 and a pressure of 1 atm controlled by the implemented Nosé–Hoover Langevin piston method with a piston period of 100 fs and a damping timescale of 50 fs. Hereafter, the membrane area was fixed, switching to the NP z AT ensemble for the remaining simulation time. Further discussion on the simulation protocol can be found in Supplementary Methods . A time step of 1 fs was used; the non-bonded interactions were calculated every second time step, and full electrostatics evaluated every fourth time step. Simulation time was 50 ns for each system. Analysis of MD simulations Descriptions of the procedures used for the analysis of the MD simulations can be found in the Supplementary Methods . Accession codes: Coordinates and experimental data for the debutanoyl thapsigargin-bound complex of rabbit sarco(endo)plasmic reticulum Ca 2+ –ATPase in the calcium-free form have been deposited in the Protein Data Bank under the accession code 2YFY . How to cite this article: Sonntag, Y. et al . Mutual adaptation of a membrane protein and its lipid bilayer during conformational changes. Nat. Commun. 2:304 doi: 10.1038/ncomms1307 (2011).